Emergence of stable polymorphisms driven by evolutionary games between mutants Under neutrality, polymorphisms are maintained through the balance between mutation and drift. Under selection, a variety of mechanisms may be involved in the maintenance of polymorphisms, for example, sexual selection or host-parasite coevolution on the population level or heterozygote advantage in diploid individuals. Here we address the emergence of polymorphisms in a population of interacting haploid individuals. In our model, each mutation generates a new evolutionary game characterized by a payoff matrix with an additional row and an additional column. Hence, in general, the fitness of new mutations is frequency-dependent rather than constant. This dynamical process is distinct from the sequential fixation of advantageous traits and naturally leads to the emergence of polymorphisms under selection. It causes substantially higher diversity than observed under the established models of neutral or frequency-independent selection. Our framework allows for the coexistence of an arbitrary number of types, but predicts an intermediate average diversity. Evolutionary dynamics is characterized by the interplay of mutation, selection and random drift [1] , [2] , [3] , [4] . Evolutionary experiments in microbes provide powerful demonstrations of all these forces at work [5] , [6] , [7] , [8] . Typically, it is assumed that mutants with a random fitness value, which remains constant throughout, arise and either go extinct or reach fixation [9] . Advantageous mutations can quickly reach fixation in the population. However, such events are too rare to substantially increase genetic diversity over time [10] , [11] , [12] . Evolutionary game theory provides an alternative perspective on evolutionary change, by modelling the fitness of a mutant as a function of the frequencies of all types of individuals in the population. For example, a mutant may be advantageous at the beginning of an invasion, but its fitness may drop below the residents' fitness when it reaches a certain abundance [2] , [4] , [13] , [14] . In such models, the number of types is usually fixed from the outset [13] , [15] . This corresponds to two (or few) allele models in population genetics [1] , [3] . Here we present a model where each mutation generates a new evolutionary game characterized by a payoff matrix with an additional row and an additional column. This represents a generalization that is analogous to the infinite-alleles model that has mainly been considered in the context of neutral or constant selection so far [3] . This approach results in substantially higher diversity than observed under the established models of neutral or frequency-independent selection and permits the coexistence of an arbitrary number of types, but predicts an intermediate average diversity. Description of the model We propose an approach where every mutation leads to a new game between the mutant and the residents. We use stochastic evolutionary game dynamics with n types of individuals in a finite population of size N (refs 16 , 17 ). Interactions between individuals are captured by an n×n payoff matrix. The payoff of a type i individual when it interacts with a type j individual is the entry a ij in the payoff matrix. The average payoff of an individual determines its fitness and is a function of the frequencies of all types. In our model, any new mutation increases the number of types in the game. We assume that mutant m inherits the payoff entries of its parent p , subject to Gaussian noise. Thus, the mutant's payoff against type j , a mj , has mean a pj , and the payoff of type j against the mutant, a jm , has mean a jp . If there are n resident types when the mutant appears, the n×n payoff matrix is extended by an additional column (the payoff entries of residents interacting with the mutant) and an additional row (the payoff entries of the mutant interacting with residents) ( Fig. 1 ). Conversely, when type j goes extinct, row j and column j in the payoff matrix are deleted, such that it is reduced to an ( n −1)×( n −1) matrix. Our reference scenario is frequency-independent (constant) selection, where each type has a fixed fitness. In this special case, each row in the payoff matrix consists of identical numbers, a ij = a ik for all i , j , and k . 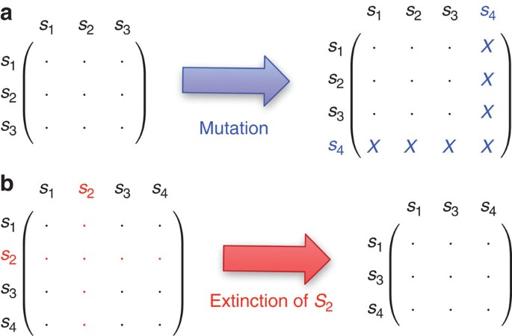Figure 1: Dynamic payoff matrices. Mutant games are characterized by growing and shrinking payoff matrices, as shown in this example with 3 and 4 types. All elements of the payoff matrix can be different, whereas for the special case of constant selection payoff entries in each row are identical. (a) A mutation increases the dimension of the payoff matrix from 3 to 4. The new column describes interactions of the previous types with the new mutant, whereas the new row describes the interactions of the new mutant with the previous types. (b) Extinction of a typeS2decreases the dimension of the payoff matrix from 4 to 3. Whenever a type goes extinct, the corresponding row and column of the payoff matrix are deleted. Figure 1: Dynamic payoff matrices. Mutant games are characterized by growing and shrinking payoff matrices, as shown in this example with 3 and 4 types. All elements of the payoff matrix can be different, whereas for the special case of constant selection payoff entries in each row are identical. ( a ) A mutation increases the dimension of the payoff matrix from 3 to 4. The new column describes interactions of the previous types with the new mutant, whereas the new row describes the interactions of the new mutant with the previous types. ( b ) Extinction of a type S 2 decreases the dimension of the payoff matrix from 4 to 3. Whenever a type goes extinct, the corresponding row and column of the payoff matrix are deleted. Full size image Mutant games between two types First, we consider the case of a single mutant B in a homogeneous population of A -types. Fitness differences depend on the distribution of payoff values and on the intensity of selection w . To avoid negative fitness values, we assume that fitness is an exponential function of the average payoff multiplied by w (see Methods ). Under constant selection with Gaussian distributed payoffs around the parent type payoff, the probability for an advantageous mutation is 50%. For frequency-dependent selection, 50% of the mutants are also initially advantageous. In 25% of the cases, the mutants' fitness is greater than that of the wild type regardless of the mutants' abundances. In these cases, the mutants will take over the population deterministically for strong selection w , or large population size N . Some of these mutations increase the average fitness and some of them will decrease it, the latter representing Prisoner's Dilemmas [13] . This game is characterized by a specific ordering of payoffs, a BA > a AA > a BB > a AB , a situation that is typically described as interactions between cooperators (type A ) and defectors (type B ). The payoff ordering implies that defectors always have higher fitness and tend to spread, but this decreases the average fitness of the population. Another 25% of the mutations are initially advantageous but lose this advantage once they become abundant and hence promote coexistence, which is reminiscent of the Hawk–Dove game [13] or the Snowdrift game [18] and characterized by the payoff ordering a BA > a AA > a AB > a BB . The remaining 50% of the mutants are disadvantageous at low frequencies and will typically be lost. However, for weak selection, w ≪ 1/ N , the stochastic nature of the process allows even slightly disadvantageous mutants to invade and fix. Conversely, advantageous mutants can also be lost for the same reason. The corresponding fixation probabilities can be calculated from a moment expansion of the distribution of payoffs [19] . Mutant games between n types Here we focus on a more general case of a continuously evolving population. New types appear and old types go extinct. No type can be fixed in the population forever. Instead of looking at the fixation probability of a certain type, we will focus on the evolutionary dynamics in such a population and see under which conditions a stable polymorphism can naturally emerge. In population genetics, frequency-dependent selection in diploids has been considered in the past, but the focus has been on special cases such as symmetric overdominance [20] , [21] . In evolutionary game theory, it is argued that frequency-dependent selection is generic, with constant selection describing a special case [2] , [14] , [16] . Our model allows us to address the consequences of frequency-dependent selection. We focus on the average number of different types simultaneously present in the population. The interactions can be any two-player game, leading to any kind of linear frequency dependence. Whereas previous models of evolutionary games with variable numbers of types were based on deterministic dynamics [22] , [23] , [24] , [25] , we focus on the more general case of stochastic evolutionary dynamics. We consider a Moran process in a population of constant size N . In every time step, one individual is randomly chosen proportional to its fitness, and produces a mutant with probability μ or an identical offspring with probability 1− μ . A randomly chosen individual in the population is replaced by this offspring. The fitness of a given individual is determined from its interactions within the population (see Methods ). Mutations increase and extinctions decrease the dimension of the payoff matrix ( Fig. 1 ). To ensure that the selection intensity is independent with evolutionary time, we normalize the payoff matrix after each mutation and after each extinction such that the highest absolute payoff value equals one. Diversities under constant selection and mutant games An example for the different dynamics arising through mutant games compared with constant selection is shown in Fig. 2 . For weak selection, Nw ≪ 1, the extinction times are of the order of N generations and frequency-dependent selection is not markedly different from constant selection. However, for larger populations or higher intensity of selection w , stable alliances can coexist for a long time [26] . Mutants can affect the population by (i) destroying existing alliances and taking over the population, (ii) enabling one of the residents or a new alliance of residents to take over or (iii) leading to another stable alliance together with a subset of the resident types or all of them. Only if the mutant type enters the population without displacing any resident, does the number of types increase. Nonetheless, frequency-dependent selection leads to a significant increase in the diversity of the population compared with neutral or constant selection. The balance between selection and drift is governed by the product of the selection intensity and the population size. For fixed selection intensity, the smaller the population, the larger the genetic drift. For fixed population size, the smaller the selection intensity, the larger the genetic drift. Here we assess the effect of genetic drift by varying the selection intensity in a population of fixed size (see Methods ). 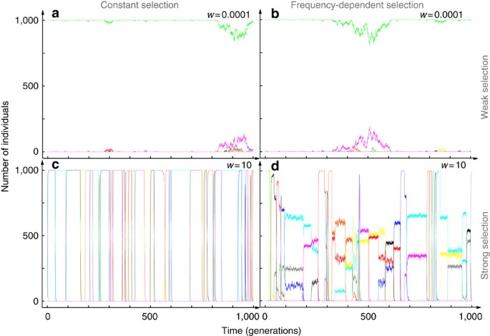Figure 2: Sample trajectories of the evolutionary dynamics in a Moran process. The left panels are for constant selection and the right panels are for frequency-dependent selection. Top: for weak selection,w=0.0001, the dynamics with constant selection (a) is similar to that with frequency-dependent selection (b), because possible coexistences disappear due to genetic drift. As on averageμ/Nmutations appear per generation,μneutral fixation events are expected per generation, and a single type dominates over 1/μgenerations. Bottom: for strong constant selection,w=10, successive fixation events of the 50% advantageous mutants are observed (c), the expected number of such events per generation isNμ/2. For frequency-dependent fitness (d), pairwise coexistences are stable over long periods of time. Additional mutants can arise and lead to the coexistence of 3 or even more types (population sizeN=1,000, mutation rateμ=10−4per time step, all simulations start from a monomorphic state). Figure 2: Sample trajectories of the evolutionary dynamics in a Moran process. The left panels are for constant selection and the right panels are for frequency-dependent selection. Top: for weak selection, w =0.0001, the dynamics with constant selection ( a ) is similar to that with frequency-dependent selection ( b ), because possible coexistences disappear due to genetic drift. As on average μ / N mutations appear per generation, μ neutral fixation events are expected per generation, and a single type dominates over 1/ μ generations. Bottom: for strong constant selection, w =10, successive fixation events of the 50% advantageous mutants are observed ( c ), the expected number of such events per generation is Nμ /2. For frequency-dependent fitness ( d ), pairwise coexistences are stable over long periods of time. Additional mutants can arise and lead to the coexistence of 3 or even more types (population size N =1,000, mutation rate μ =10 −4 per time step, all simulations start from a monomorphic state). Full size image To further analyse diversity, let us recall population genetics under weak selection. Under neutrality and low mutation, the average number of different types, which can sometimes increase by mutation and always decreases by extinction, is described by Ewens' sampling formula [27] (see Methods ). To ensure that there can be an equilibrium between mutations and extinctions, we must assume μ ≪ N −1 . In large populations, this condition is violated and the diversity is substantially higher. Even in this case, frequency-dependent selection leads to more diversity than constant selection (see Methods ). Our weak selection results recover Ewens' sampling formula, both under constant and frequency-dependent selection. However, for strong selection, the results are strikingly different in these two cases. For constant selection, diversity decreases with increasing intensity of selection, because the extinction and fixation times become shorter. In contrast, increasing the selection intensity under frequency-dependent selection stabilizes alliances between different types and typically increases diversity ( Fig. 3 ). For small mutation rates, μ ≪ N −2 , neutral mutations go extinct on a faster timescale than new mutations arise, but polymorphisms may still exist for a long time. Mutations lead to transitions between monomorphic states or coexistence states involving 2,3,4 or more types under strong selection ( Fig. 4 ). The stationary distribution of these coexistence states can be computed based on the transition probabilities (see Methods ). This recovers our results for the distribution of the number of coexisting types ( Fig. 3 ). Evolutionary dynamics selects stable polymorphisms, but diversity is an emergent property because our mutant games lead to all possible payoff matrices. 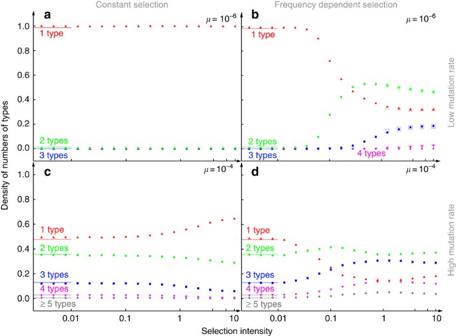Figure 3: Distribution of the number of types. The probability of observing a certain number of coexisting types is shown for different selection intensities. As expected, our simulations (filled symbols) agree with Ewens' sampling formula under weak selection (lines). The top panels show a low mutation rate,μ=10−6per time step. For constant selection (a), diversity decreases slightly with increasing intensity of selection. For frequency-dependent selection (b), diversity increases substantially with increasing intensity of selection. For strong selection, we can alternatively compute the stationary distribution from the transitions between the different polymorphisms (Fig. 3(open symbols)). Although the number of types is not limited in our model, there are typically 4 or less types coexisting in our simulations at the same time. The bottom panels show higher mutation rates,μ=10−4per time step, where the diversity under neutral selection is already high. Under frequency-independent selection (c) diversity increases compared with (a), owing to the increasing mutation rate. But frequency-dependent selection (d) increases diversity further compared with constant fitness (c) or lower mutation rates (b) (population sizeN=1,000, averages obtained over 500 independent realizations and 107generations per realization. All simulations begin in a monomorphic state, averages start after 25,000 generations). Figure 3: Distribution of the number of types. The probability of observing a certain number of coexisting types is shown for different selection intensities. As expected, our simulations (filled symbols) agree with Ewens' sampling formula under weak selection (lines). The top panels show a low mutation rate, μ =10 −6 per time step. For constant selection ( a ), diversity decreases slightly with increasing intensity of selection. For frequency-dependent selection ( b ), diversity increases substantially with increasing intensity of selection. For strong selection, we can alternatively compute the stationary distribution from the transitions between the different polymorphisms ( Fig. 3 (open symbols)). Although the number of types is not limited in our model, there are typically 4 or less types coexisting in our simulations at the same time. The bottom panels show higher mutation rates, μ =10 −4 per time step, where the diversity under neutral selection is already high. Under frequency-independent selection ( c ) diversity increases compared with ( a ), owing to the increasing mutation rate. But frequency-dependent selection ( d ) increases diversity further compared with constant fitness ( c ) or lower mutation rates ( b ) (population size N =1,000, averages obtained over 500 independent realizations and 10 7 generations per realization. All simulations begin in a monomorphic state, averages start after 25,000 generations). 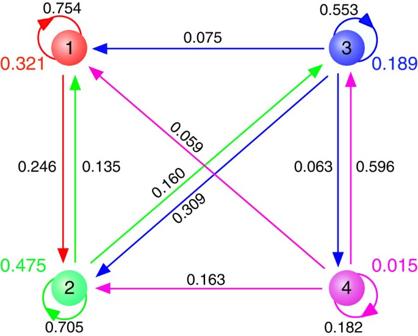Figure 4: Transition probabilities between different levels of diversity. The consequences of mutations for the diversity are described by transition probabilities for low mutation rates under strong selection. The transition probability between different levels of diversity results from the appearance of a mutant. Each circle marks a certain number of coexisting types and the probability that the population is in this state (cf. toFig. 3b), arrows mark the probabilities of the transitions between these states after the appearance of a mutant. A mutation can only increase the diversity by at most one type, but this probability decays rapidly with the number of coexisting types. A new mutation can also lead to a decrease in the diversity to any level. Here we show the transitions for up to four coexisting types under strong selection; as illustrated inFig. 3b, the probability to be in states withn>4 under strong selection is negligible for the present parameter combination. (population sizeN=1,000, mutation rateμ=10−6per time step, selection intensityw=10, averages obtained over 500 independent realizations and 107generations per realization after a transient period of 25,000 generations. All simulations start from a monomorphic state). Full size image Figure 4: Transition probabilities between different levels of diversity. The consequences of mutations for the diversity are described by transition probabilities for low mutation rates under strong selection. The transition probability between different levels of diversity results from the appearance of a mutant. Each circle marks a certain number of coexisting types and the probability that the population is in this state (cf. to Fig. 3b ), arrows mark the probabilities of the transitions between these states after the appearance of a mutant. A mutation can only increase the diversity by at most one type, but this probability decays rapidly with the number of coexisting types. A new mutation can also lead to a decrease in the diversity to any level. Here we show the transitions for up to four coexisting types under strong selection; as illustrated in Fig. 3b , the probability to be in states with n >4 under strong selection is negligible for the present parameter combination. (population size N =1,000, mutation rate μ =10 −6 per time step, selection intensity w =10, averages obtained over 500 independent realizations and 10 7 generations per realization after a transient period of 25,000 generations. All simulations start from a monomorphic state). Full size image The nature of the games As soon as more than two types coexist, we can also analyse the interactions of each pair of types. Here we focus on 2×2 subgames of the observed 3×3 games. As a polymorphism of n types usually arises from a previous polymorphism of n −1 types, the vast majority of the 2×2 subgames ( ∼ 90%) show stable coexistences. However, there is a small fraction of 2×2 games in which one type dominates over the other. In particular, when viewed in isolation, a few of these pairs engage in Prisoner's Dilemma interactions ( ∼ 1%). Despite the metaphorical power of the Prisoner's Dilemma in the theory of evolution of cooperation, there is a striking lack of empirical cases described by this model [28] . The relative rarity of Prisoner's Dilemma relationships occurring in mutant games seems to corroborate the dearth of empirical evidence for it. Besides, restricting the analysis to pairwise interaction in this way can be misleading, because any pair of individuals represents just a subset of a more complex interacting community of many types. For example, they could be part of a rock-scissors-paper-type cyclic dominance hierarchy that is known for its capacity to support coexistence [29] , [30] . In contrast, ∼ 10% of pairwise interactions represent Snowdrift games, which do not mandate the presence of further types or other mechanisms to account for polymorphisms. Hence the Snowdrift game seems a biologically appealing and possibly more relevant framework to address cooperation [18] . Complex communities can only be observed when the intensity of selection is strong, which means that the rate of adaptation of a population to external conditions is relatively high. HIV evolution, host-parasite coevolution, or antibiotic resistance are examples for high selective pressures. Moreover, intraclonal polymorphism is frequently observed in bacterial species [31] , [32] . Our mutant games show an intriguing resemblance to recent observations in long-term evolutionary experiments with Escherichia coli : When kept in a constant environment, these bacteria alternate between monomorphic phases and coexistence of up to a handful of distinct genotypes for hundreds of generations [32] , similar to our strong selection case in Fig. 2 . Frequency-dependent selection is a recurrent theme in evolutionary biology, with applications as diverse as Fisher's explanation of the 1:1 sex ratios [33] , sympatric speciation [34] , and the allelic diversity of the immune system driven by host parasite coevolution [35] . In each case, the most important consequences for the evolutionary process arise through frequency dependence and, in particular, through stable polymorphisms. In our model, any mutation produces a new game between mutant type and resident types, which takes the full spectrum of frequency dependence into account. It is straightforward to extend our framework to diploid populations, where pairwise games correspond to the interactions of two alleles at one locus [21] (see Methods ), and frequency-dependent selection arises from diploidy rather than interaction between different genotypes. Under constant selection, the average fitness of a population keeps increasing (neglecting occasional dips due to the stochastic fixation of disadvantageous mutants), which contrasts with the proposed mutant games where frequency-dependent selection may result in an increase as well as a decrease of fitness. Evolutionary processes represent an optimization to a changing environment [14] , but in addition, evolutionary trajectories are constrained through inheritance and mutations. Mutant games capture all these effects in a concise framework and present a complementary perspective on the emergence of polymorphisms and the degree of diversity. Payoff and fitness In evolutionary game theory, the fitness of individuals is determined through games, that is, interactions with other individuals. In our case, the game is characterized by a payoff matrix. If only two types, S 1 and S 2 , interact, the payoff matrix is given by In our model, the payoff is determined from interactions with all other individuals in the population, excluding self interactions. Thus, the payoff of type S 1 is where i is the number of S 1 individuals in the population. Equivalently, we have for the payoff of type S 2 . To avoid the complications of negative fitness, we define the fitness, f j , of type j as an exponential function of its payoff π j , Here w (0≤ w <∞) controls the selective differences between players with different payoffs [36] . If a 11 = a 12 , and a 21 = a 22 , the payoffs are independent of interactions and are only determined by the type of the individuals. This special case corresponds to constant selection, where the fitness of one type does not depend on the frequency of the types in the population. Neutral selection corresponds to w =0 or to a 11 = a 21 = a 12 = a 22 . In a population of n types, we use a n × n matrix to describe the payoffs. When a mutant appears, an additional column and row are added to the matrix to describe the additional interactions. In the general frequency-dependent case, 2 n +1 new payoff matrix entries have to be defined. In contrast, for constant selection, only one new variable is needed to describe the fitness of a mutant. There are several ways to generate these new variables. Suppose that m is the mutant type, j is a resident type, and p is the mutant's parent type. In the simplest case, the payoffs of the mutant m against the resident types j , a mj , and the payoffs of the resident types against the new mutant, a jm , are chosen randomly and independently of the current types from some probability distributions. But it is more natural, if the mutants are similar to their parents by inheriting some aspects of their payoff entries. To this end, we randomly choose the payoff of the mutant against a certain resident from a distribution around its parent's payoff against that resident. Although we can take arbitrary distributions for the payoff entries in our model, we focus on the simplest case, where the payoff entries of the offspring are Gaussian distributed around its parent's payoff entries. In other words, the mean of the new payoff entries a mj for the mutant m is given by the payoff a pj of its parent type p against a type j individual. An equivalent rule holds for the payoff of the resident types against a mutant, the new payoff entries a jm have mean a jp . For the Gaussian distribution, a change in the variance corresponds to a change in the intensity of selection [19] . Thus, we always set the variance to one. This approach implies that mutations with selective advantage are favoured, such that the average fitness increases over time. In our case, this would mean that the effective intensity of selection is also increasing, making the system nonstationary. To avoid this effect, we rescale the payoff matrix by dividing it by the largest absolute value of all payoff entries after every mutation and every extinction. With the full information on the payoffs, we can calculate the fitness of all types in the population based on the payoff matrix. For example, type j obtains the payoff where i k is the number of type k individuals in the population and d is the number of types. Moran dynamics The Moran process describes the evolutionary dynamics in a finite population with overlapping generations [16] , [36] , [37] . We start with a homogeneous population with constant size N =1,000 and payoff a 11 =1. In every time step, one individual is chosen randomly in proportion to its fitness, and produces an identical offspring with probability 1− μ or a mutant with probability μ . The offspring then replaces a randomly chosen individual. In nature, mutation rates can range from 10 −8 to 10 −3 per base, per generation [38] . Although mutation rates are not affected by local population size, the effect of mutation rates on diversity is directly related to it. To investigate realistic mutation rates in our model, we consider it based on the population size N . As our primary interest is diversity driven by selection rather than diversity driven by mutations, we focus on low mutation rates here. When the mutation rate is high, μ >1/ N , the differences between the population dynamics under frequency-dependent and constant selection are less obvious, as the diversity is mainly driven by mutation. In the case of μ =1/ N , frequency-dependent selection still leads to higher diversity, compared with constant selection ( Supplementary Fig. S1 ). In either case diversity tends to decrease for strong selection, which becomes more pronounced for higher mutation rates ( Fig. 3; Supplementary Fig. S1 ). The reason is that there are only relatively few coexistence games and mutant types may destabilize them—and the stronger the selection, the faster this occurs. When a mutation occurs, we generate the payoff matrix according to the method described above. We record the number of individuals of different types in every time step, which gives a straightforward picture of the population dynamics over time. As the system evolves for a long time, we record the number of types in every generation. To avoid dependence on the initial condition, we excluded the data of the first 25,000 generations (see the captions of figures) in the averages. To compare constant fitness and frequency-dependent fitness, we run simulations in both cases, which only differ in the process for generating payoff matrices. The results under weak selection reflect the usual statistical properties of genetic data samples. The probability of m different alleles present in the population under neutral selection, P ( m ), can be calculated by Ewens' sampling formula, , where are the unsigned Stirling numbers of the first kind [3] , [39] . For a haploid Moran process, as in our case, the parameter θ is Nμ . Transition probabilities between different coexistence states Let us consider selection scenarios generated by introducing mutants. Under strong selection and low mutation rates, a population is usually in an equilibrium where different types coexist with each other. The appearance of a new mutant during a phase of coexistence can lead to establishment of a new alliance with the new mutant as an additional type, formation of a new alliance with fewer types (which may include the mutant type or not), replacement of one type from the previous alliance with the new mutant, or extinction of the mutant. Here we infer the probabilities of these selective consequences under the Moran process. We assume a mutation rate μ ≪ N −2 . In this case, the average time of waiting for a new mutant is much longer than the average time a population needs to reach a new equilibrium after a mutation. We start simulations from a homogeneous population. Mutants show up at random. After a mutant appears, we wait until the population reaches a new equilibrium, and infer whether the diversity has decreased, increased or been maintained. Each state is characterized only by the number of coexisting types. For example, state one represents that the population is homogeneous, and state two represents that there are two types coexisting. We are interested in the probability that a population changes from one state to another. The transition matrix between different states T is obtained by averaging over the evolutionary trajectories. The element t ij denotes the transition probability from i to j coexisting types. For low mutation rates, t ij is very small for j>i +1. The fraction of time that the population spends in each state of diversity is then given by the stationary distribution of the Markov chain determined by the transition matrix T ( Fig. 4 ). Population size For fixed selection intensity, the smaller the population size is, the larger the genetic drift. For fixed population size, the smaller the selection intensity is, the larger the genetic drift. Thus, the stochastic effect from the small population size is similar to a smaller intensity of selection. Instead of having two parameters that lead to the same effect, we focussed our discussion on the case of N =1,000 for various intensities of selection. Focussing on variable selection intensities is computationally less costly than varying the population size. For both the Moran process and the Wright–Fisher process, the required CPU time scales with the population size, but not with the intensity of selection. For comparison, we also carried out simulations for N =100, where the same patterns of difference between frequency-dependent selection and constant selection are observed ( Supplementary Fig. S2 ). Diploid populations The evolutionary game dynamics for Mendelian populations has been studied in detail in the past [40] , [41] , [42] ; the interaction of two alleles at a diploid locus can be interpreted as a special kind of two-player game, which has a symmetric payoff matrix [43] , [44] , [45] . Suppose there are two types of alleles, allele A and allele B. The fitness of a homozygous individual AA is w AA , the fitness of a BB individual is w BB and the fitness of a heterozygous individual AB is w AB . This can be formalized as When w AA > w AB and w BB > w AB , it corresponds to under-dominance, where heterozygous individuals have a lower fitness than homozygous individuals. When w AA < w AB and w BB < w AB , a condition of over-dominace is described. A diploid population with more than two types of alleles at a single locus can be described by a symmetric n × n matrix, where n is the number of different alleles and matrix element w ij represents the fitness of a diploid individual with genotype ij . We have simulated the dynamics of such a diploid population under different selection intensities based on the Moran process ( Supplementary Fig. S3 ). In every time step, one allele is replaced, and thus the time for one generation is twice as long as the one in a haploid Moran model. Under the same mutation rate, the diversity of a diploid population ( Supplementary Fig. S3a ) is higher compared with the frequency-dependent case in a haploid population ( Fig. 4b ). This is because symmetry of the payoff matrix w ij = w ji favours coexistence of different types. In the simplest case with only two alleles, a coexistence game corresponding to over-dominance has the ordering of payoffs, w AA < w AB and w BB < w AB . Suppose allele A is a random mutant from allele B , and the payoffs of the new genotypes, w BB and w AB , are random variables with mean w BB . Thus, the probability to have a coexistence of these two alleles is 37.5%, which is larger than 25%, the probability to have a coexistence in a two-allele haploid model. In the diploid approach, the fitness of a genotype ij , w ij , is a constant number, and does not change with the composition of the frequencies of different genotypes (but the fitness of an allele is frequency dependent). Hence, this kind of frequency dependence corresponds to constant selection in a haploid population. To introduce frequency dependence on this level leads to serious mathematical intricacies [40] , [43] , [45] , [46] . Wright-Fisher dynamics In the Wright-Fisher Model, all individuals produce a large number of offspring proportional to their fitness. Then, all individuals from the previous generation die, and are replaced by N new individuals sampled at random from the offspring pool. This corresponds to a multinomial sampling of offspring. The expected number of offspring of a certain type, j , in the next generation is proportional to its fitness. Neglecting mutations, the expected number of type j is where, i j and f j are the number of individuals and the fitness of type j . If there is no difference in fitness between types in the population, the expected number of individuals of the different types is constant and the composition of the population will only be changed by random drift. When we consider mutations, the probability that an offspring mutates is μ . On average, there are Nμ new mutants in the population per generation. We analyse the same quantities in the Wright–Fisher process as above in the Moran process. We see similar patterns in the differences between constant selection and frequency-dependent selection ( Supplementary Fig. S4 ). However, for very strong selection, diversity decreases in our set-up. This can be understood as follows: consider a stable coexistence between two types. If a fluctuation leads the system away from this point, one type has a slight payoff advantage, which causes a large fitness advantage owing to our exponential payoff to fitness mapping. Such a fluctuation can lead to the immediate fixation of one type in the next generation and thus destroy the stable coexistence quickly. Again, under weak selection and low mutation rates, we recover the diversity given by Ewens' sampling formula. Under neutral selection, random drift in a Moran process is twice as strong as in a Wright–Fisher process [47] . Thus, we have θ =2 Nμ in Ewens' sampling formula for the Wright–Fisher process. How to cite this article: Huang, W. et al . Emergence of stable polymorphisms driven by evolutionary games between mutants. Nat. Commun. 3:919 doi: 10.1038/ncomms1930 (2012).